An atlas of DNA methylomes in porcine adipose and muscle tissues It is evident that epigenetic factors, especially DNA methylation, have essential roles in obesity development. Here, using pig as a model, we investigate the systematic association between DNA methylation and obesity. We sample eight variant adipose and two distinct skeletal muscle tissues from three pig breeds living within comparable environments but displaying distinct fat level. We generate 1,381 Gb of sequence data from 180 methylated DNA immunoprecipitation libraries, and provide a genome-wide DNA methylation map as well as a gene expression map for adipose and muscle studies. The analysis shows global similarity and difference among breeds, sexes and anatomic locations, and identifies the differentially methylated regions. The differentially methylated regions in promoters are highly associated with obesity development via expression repression of both known obesity-related genes and novel genes. This comprehensive map provides a solid basis for exploring epigenetic mechanisms of adipose deposition and muscle growth. Obesity can be considered an epidemic that has become a major threat to the quality of human life in modern society [1] . By 2030, up to 58% of the world's adult population might be either overweight or obese [1] . Adipose tissues (ATs) and skeletal muscle tissues (SMTs) have important roles in the pathogenesis of obesity and its comorbidities by secreting cytokines involved in the regulation of metabolism [2] , [3] . The metabolic risk factors of obesity and increased body weight are more related to adipose distribution rather than the total adipose mass [4] , [5] . ATs located within the abdominal and thoracic cavity, known as visceral ATs (VATs), have been recognised to be anatomically, functionally and metabolically distinct from that of the compartmental subcutaneous ATs (SATs) [6] , and have been found to be related to a series of diseases, including cardiovascular disease, type II diabetes mellitus and metabolic syndrome [7] . Nonetheless, SATs can have direct and beneficial effects on the control of body weight and metabolism [8] . Pig ( Sus scrofa ) is emerging as an attractive biomedical model for studying energy metabolism and obesity in humans, because of their similar metabolic features, cardiovascular systems, proportional organ sizes and lack of brown adipose postnatally [9] . The pig model offers, in fact, the advantages of low genetic variance, homogeneous feeding regime and remitting confounding factors typical of humans, such as smoking, alcohol drinking and so on. In the modern industry, pigs have undergone strong genetic selection in the relatively inbred commercial lines for lean meat production, or in some cases, for adipose production, which has led to remarkable phenotypic changes and genetic adaptation, making these breed lines a perfect model for comparative studies [10] , [11] . There has been extensive research to hunt for 'obesity alleles', most recently by whole-genome association studies [12] , [13] . It is evident that DNA sequence polymorphism alone does not provide adequate explanations for mechanisms of obesity regulation. Recently, epigenetic factors, especially DNA methylation that is a stably inherited modification affecting gene regulation and cellular differentiation, has gained a greater appreciation as an alternative perspective on the aetiology of complex diseases [14] , [15] . Nevertheless, current understanding of the roles of DNA methylation in the aetiology of obesity remains fairly rudimentary [16] . Here, for three well-defined pig breeds displaying distinct fat contents in comparable environments, we collected eight ATs from different body sites and two phenotypically distinct SMTs, and studied genome-wide DNA methylation differences among breeds, sexes and anatomic locations. We showed the landscape of methylome distribution in the genome, analysed differentially methylated regions (DMRs) and identified genes that were involved in the development of obesity. The work performed here will serve as a valuable resource for future functional validation and aid in searching for epigenetic biomarkers for obesity prediction and prevention, and promoting further development of pig as a model organism for human obesity research. Samples and their obesity-related phenotypes We chose three pig breeds in this study, based on known history of breed formation and measurement of obesity-related phenotypes (see Supplementary Methods ). The Landrace breed has been selected for less adipose for more than 100 years in Europe, whereas the Rongchang breed was selected for extreme adipose. The Tibetan breed is almost a feral breed that has undergone very little artificial selection. On average, adult females exhibit higher fat percent than males upon reaching sexual maturity at 210 days old. To investigate sexual differences, we also separated males and females in the comparison. As expected, body density, which negatively correlates with fat percent, showed significant difference among the three breeds (two-way analysis of variance (ANOVA), P B =6.98×10 −10 ) and between male and female (two-way ANOVA, P S =0.02; Fig. 1a ). Measurement of metabolism indicators in serum also revealed the same ranking ( Supplementary Fig. S1 ). 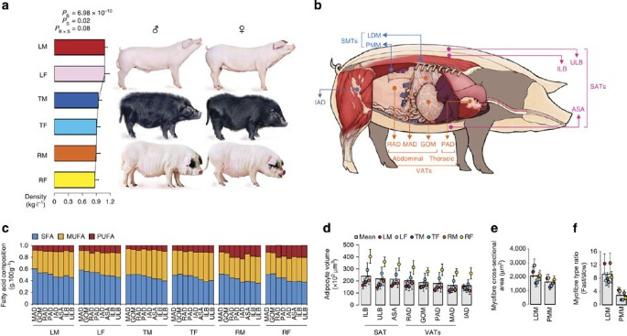Figure 1: Characteristics of pig ATs and SMTs. (a) Body density difference among Landrace (L), Tibetan (T) and Rongchang (R) pigs, and between male (M) and female (F). Two-way repeated-measures ANOVA (n=9 per breed per sex). 'B' and 'S' mean breed and sex, respectively. Values are means±s.d. (b) Sources of tissues: three SATs (ASA: abdominal subcutaneous adipose, ILB: inner layer of backfat, ULB: upper layer of backfat), four VATs (GOM: greater omentum, MAD: mesenteric adipose, RAD: retroperitoneal adipose, PAD: pericardial adipose), intermuscular adipose (IAD) and two SMTs (LDM:longissimus dorsimuscle, and PMM:psoasmajor muscle). (c) Fatty acid composition difference. SFA, MUFA and PUFA mean saturated, monounsaturated, and polyunsaturated fatty acid, respectively. Three-way repeated-measures ANOVA (n=9 per breed per sex per tissue). (SFA:PB=2.46×10−7,PS=1.35×10−6,PT=0.99,PB×S=0.19,PB×T=0.96,PS×T=0.69,PB×S×T=0.77; MUFA:PB=0.006,PS=0.0004,PT=0.98,PB×S=0.99,PB×T=0.99,PS×T=0.93,PB×S×T=0.77; and PUFA:PB=0.0008,PS=0.14,PT=0.98,PB×S=0.03,PB×T=0.99,PS×T=0.56,PB×S×T=0.099). (d) Adipocyte volume difference. Three-way repeated-measures ANOVA (n=9 per breed per sex per tissue). 'T' means tissue. (PB<10−16,PS=10−16,PT=6.74×10−12,PB×S<10−16,PB×T=0.29,PS×T=0.36,PB×S×T=0.99). Values are means±s.d. (e) Myofibre cross-sectional area difference. Three-way repeated-measures ANOVA (n=9 per breed per sex per tissue;PB<10−16,PS=0.005,PT=9.66×10−12,PB×S=0.44,PB×T=0.01,PS×T=0.583,PB×S×T=0.07). (f) Myofibre type ratio difference. Three-way repeated-measures ANOVA (n=9 per breed per sex per tissue;PB=4.42×10−10,PS=5.45×10−9,PT<10−16,PB×S=0.004,PB×T=0.02,PS×T=1.61×10−5,PB×S×T=0.04). Figure 1: Characteristics of pig ATs and SMTs. ( a ) Body density difference among Landrace (L), Tibetan (T) and Rongchang (R) pigs, and between male (M) and female (F). Two-way repeated-measures ANOVA ( n =9 per breed per sex). 'B' and 'S' mean breed and sex, respectively. Values are means±s.d. ( b ) Sources of tissues: three SATs (ASA: abdominal subcutaneous adipose, ILB: inner layer of backfat, ULB: upper layer of backfat), four VATs (GOM: greater omentum, MAD: mesenteric adipose, RAD: retroperitoneal adipose, PAD: pericardial adipose), intermuscular adipose (IAD) and two SMTs (LDM: longissimus dorsi muscle, and PMM: psoas major muscle). ( c ) Fatty acid composition difference. SFA, MUFA and PUFA mean saturated, monounsaturated, and polyunsaturated fatty acid, respectively. Three-way repeated-measures ANOVA ( n =9 per breed per sex per tissue). (SFA: P B =2.46×10 −7 , P S =1.35×10 −6 , P T =0.99, P B×S =0.19, P B×T =0.96, P S×T =0.69, P B×S×T =0.77; MUFA: P B =0.006, P S =0.0004, P T =0.98, P B×S =0.99, P B×T =0.99, P S×T =0.93, P B×S×T =0.77; and PUFA: P B =0.0008, P S =0.14, P T =0.98, P B×S =0.03, P B×T =0.99, P S×T =0.56, P B×S×T =0.099). ( d ) Adipocyte volume difference. Three-way repeated-measures ANOVA ( n =9 per breed per sex per tissue). 'T' means tissue. ( P B <10 −16 , P S =10 −16 , P T =6.74×10 −12 , P B×S <10 −16 , P B×T =0.29, P S×T =0.36, P B×S×T =0.99). Values are means±s.d. ( e ) Myofibre cross-sectional area difference. Three-way repeated-measures ANOVA ( n =9 per breed per sex per tissue; P B <10 −16 , P S =0.005, P T =9.66×10 −12 , P B×S =0.44, P B×T =0.01, P S×T =0.583, P B×S×T =0.07). ( f ) Myofibre type ratio difference. Three-way repeated-measures ANOVA ( n =9 per breed per sex per tissue; P B =4.42×10 −10 , P S =5.45×10 −9 , P T <10 −16 , P B×S =0.004, P B×T =0.02, P S×T =1.61×10 −5 , P B×S×T =0.04). Full size image To study adipocyte regulation in different anatomic locations, we sampled eight ATs from various body regions ( Fig. 1b ), which exhibited dissimilar fatty acid composition ( Fig. 1c ) and significantly different adipocyte volumes (three-way ANOVA, P T =6.74×10 −12 ) among the three breeds (three-way ANOVA, P B <10 −16 ), and between males and females (three-way ANOVA, P S =10 −16 ; Fig. 1d ; Supplementary Fig. S2 ). We also sampled two SMTs, white longissimus dorsi muscle (LDM) and red psoas major muscle (PMM; Fig. 1b ), representing two different fibre types, of which PMM has a higher percentage of capillaries, myoglobin, lipids and mitochondria [17] . Compared with PMM, LDM has higher myofibre cross-sectional area (three-way ANOVA , P T =9.66×10 −12 ; Fig. 1e ; Supplementary Fig. S2 ) and ratio of fast to slow twitch myofibre (three-way ANOVA , P T <10 −16 ; Fig. 1f ; Supplementary Fig. S2 ). There is also significant divergence in myofibre cross-sectional area (three-way ANOVA , P B <10 −16 , P S =0.005) and myofibre type ratio (three-way ANOVA, P B =4.42×10 −10 , P S =5.45×10 −9 ) among the three breeds and between the two sexes. These phenotypic differences for ATs and SMTs between breeds, sexes and anatomic locations imply the intrinsically epigenomic differences. Landscape of the DNA methylomes We generated a total of 1,381 Gb methylated DNA immunoprecipitation sequencing (MeDIP-seq) data from 180 samples (~7.67 Gb per sample), of which 1,067 Gb (77.3%) clean reads were aligned on the pig genome. After removing the ambiguously mapped reads and reads that may have come from duplicate clones, we used 993 Gb (71.9%) uniquely aligned non-duplicate reads in the following analysis ( Supplementary Table S1 ). To avoid false positives in enrichment, we required at least ten reads to determine a methylated CpG in a sample. On average, 16.1% of the CpGs were covered by this threshold ( Supplementary Fig. S3 ). Measurement of DNA methylation level along chromosomes showed that the X chromosome is globally hypermethylated in females compared with males ( Fig. 2a ), which can be explained by the X chromosome inactivation in females [18] . Through comparison of DNA methylation level between each pair of samples, we found variable correlation rates in different categories ( Fig. 2b ). The biological replicates highly correlated with each other (median Pearson's r =0.95 for SMTs and r =0.94 for ATs), which suggested both experimental reliability and epigenetic consistency within the same breed/sex/tissue type group. The correlation rates were relatively lower between male and female (median Pearson's r =0.92 for SMTs and r =0.91 for ATs), and even lower between different anatomic locations (median Pearson's r =0.91 for SMTs, r =0.89 for between ATs and SMTs, and r =0.87 for ATs) and between different breeds (median Pearson's r =0.88 for ATs and r =0.84 for SMTs), indicating significant biological differences in the latter categories. 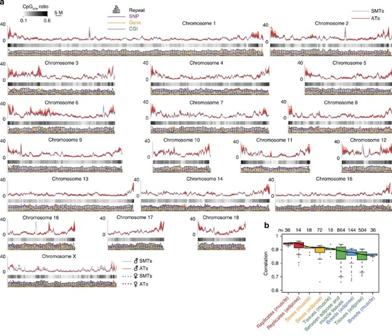Figure 2: Chromosomal profiles of pig ATs and SMTs methylomes and their variability. (a) Distribution of DNA methylation level on the pig genome. To compare DNA methylation rates among samples, read depth was normalised by overall average amount of reads in each group, and then a 1 Mb sliding window was used to smooth the distribution. The CpGo/eratio, density of SNP, gene, repeat and CGI were all calculated by 1 Mb sliding window. (b) Boxplots of pairwise Pearson's correlation on methylation rate between samples. The correlation rate between every two samples was calculated by 1 kb sliding window. Then these correlation rates were grouped into the following categories: biological replicates, the same sex, the same tissues, the same breeds and between adipose and muscle tissues. As X chromosome has obviously higher methylation level in female than in male, we excluded it in the analysis between sexes. Boxes denote the interquartile range (IQR) between the first and third quartiles (25th and 75th percentiles, respectively) and the line inside denotes the median. Whiskers denote the lowest and highest values within 1.5 times IQR from the first and third quartiles, respectively. Outliers beyond the whiskers shown as black dots. Figure 2: Chromosomal profiles of pig ATs and SMTs methylomes and their variability. ( a ) Distribution of DNA methylation level on the pig genome. To compare DNA methylation rates among samples, read depth was normalised by overall average amount of reads in each group, and then a 1 Mb sliding window was used to smooth the distribution. The CpG o/e ratio, density of SNP, gene, repeat and CGI were all calculated by 1 Mb sliding window. ( b ) Boxplots of pairwise Pearson's correlation on methylation rate between samples. The correlation rate between every two samples was calculated by 1 kb sliding window. Then these correlation rates were grouped into the following categories: biological replicates, the same sex, the same tissues, the same breeds and between adipose and muscle tissues. As X chromosome has obviously higher methylation level in female than in male, we excluded it in the analysis between sexes. Boxes denote the interquartile range (IQR) between the first and third quartiles (25th and 75th percentiles, respectively) and the line inside denotes the median. Whiskers denote the lowest and highest values within 1.5 times IQR from the first and third quartiles, respectively. Outliers beyond the whiskers shown as black dots. Full size image We observed that methylation level correlates negatively with chromosome length (Pearson's r =−0.614, P =0.005) and positively with GC content (Pearson's r =0.784, P =7×10 −5 ), repeat density (Pearson's r =0.336, P =0.159), gene density (Pearson's r =0.535, P =0.018), and especially with observed over expected number of CpG (CpG o/e ) ratio (Pearson's r =0.902, P =1.33×10 −7 ) ( Fig. 3a ), which is consistent with previous reports [19] . More detailed analysis showed that the regions with GC content around 46% and CpG o/e ratio around 0.35 tend to have a higher methylation level ( Fig. 3b,c ), where the average GC content in the pig genome is 40% and CpG o/e ratio is 0.21 ( Fig. 3d,e ). Nonetheless, there is no significant correlation between the GC content and CpG o/e ratio on a genomic scale (Pearson's r =0.10, P =0.106; Fig. 3f ). The analysis showed that CpG o/e ratio has a higher correlation rate with DNA methylation level than with GC content. Single-nucleotide polymorphism (SNP) density also positively correlated with the methylation level (Pearson's r =0.597, P =0.007; Fig. 3a ). Although substantial association of SNP density and DNA methylation level has been found [20] , the mechanism is still unclear. Furthermore, the gene-rich subtelomeric region (7 Mb from each telomere) has significantly higher methylation in most (~80%, 15 out of 19) chromosomes (Student's t -test, P <0.01; Fig. 3g ). 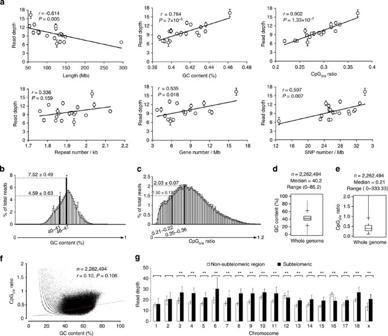Figure 3: DNA methylation level with genomic features. (a) The Pearson's correlation between DNA methylation level and features of pig autosomes (chromosomes 1–18) and sex chromosome X. The read depth was plotted against the length, GC content, repeat density, gene density, CpGo/eratio and SNP density of individual chromosome. Line represents linear regression. Values are means±s.d (n=180). (b–e) Sequencing reads distribution against CpGo/eratio and GC content. Reads distribution against (b) GC content and (c) CpGo/eratio over all samples. Values are means±s.d (n=180). Box plot of (d) GC content and (e) CpGo/eratio of the whole genome in 1 kb windows. Boxes denote the interquartile range (IQR) between the first and third quartiles (25th and 75th percentiles, respectively) and the line inside denotes the median. Whiskers denote the lowest and highest values within 1.5 times IQR from the first and third quartiles, respectively. Outliers beyond the whiskers shown as black dots. The 46–47% GC content and 0.35–0.36 CpGo/eratio are corresponding to the maximal % of total reads, that is, 7.52±0.49 and 2.03±0.07%, respectively. The genomic median of GC content (40–41%) and CpGo/eratio (0.21–0.22) are corresponding to 4.59±0.63 and 1.50±0.17% of total reads, respectively. (f) GC content versus CpGo/eratio plot of 1 kb windows across the pig genome. The pig genome was divided into 2,262,494 windows of 1 kb, and the windows were used to calculate the Pearson's correlation coefficient (r) between the GC content and CpGo/eratio. Red line represents linear regression. (g) Methylation levels in subtelomeric (up to 7 Mb from each telomere) and non-subtelomeric regions in each chromosome. (Student'st-test, **P<0.01). Values are means±s.d (n=180). Figure 3: DNA methylation level with genomic features. ( a ) The Pearson's correlation between DNA methylation level and features of pig autosomes (chromosomes 1–18) and sex chromosome X. The read depth was plotted against the length, GC content, repeat density, gene density, CpG o/e ratio and SNP density of individual chromosome. Line represents linear regression. Values are means±s.d ( n =180). ( b – e ) Sequencing reads distribution against CpG o/e ratio and GC content. Reads distribution against ( b ) GC content and ( c ) CpG o/e ratio over all samples. Values are means±s.d ( n =180). Box plot of ( d ) GC content and ( e ) CpG o/e ratio of the whole genome in 1 kb windows. Boxes denote the interquartile range (IQR) between the first and third quartiles (25th and 75th percentiles, respectively) and the line inside denotes the median. Whiskers denote the lowest and highest values within 1.5 times IQR from the first and third quartiles, respectively. Outliers beyond the whiskers shown as black dots. The 46–47% GC content and 0.35–0.36 CpG o/e ratio are corresponding to the maximal % of total reads, that is, 7.52±0.49 and 2.03±0.07%, respectively. The genomic median of GC content (40–41%) and CpG o/e ratio (0.21–0.22) are corresponding to 4.59±0.63 and 1.50±0.17% of total reads, respectively. ( f ) GC content versus CpG o/e ratio plot of 1 kb windows across the pig genome. The pig genome was divided into 2,262,494 windows of 1 kb, and the windows were used to calculate the Pearson's correlation coefficient ( r ) between the GC content and CpG o/e ratio. Red line represents linear regression. ( g ) Methylation levels in subtelomeric (up to 7 Mb from each telomere) and non-subtelomeric regions in each chromosome. (Student's t -test, ** P <0.01). Values are means±s.d ( n =180). Full size image Characterisation of DMRs We used statistics to measure the methylation rate changes and defined DMRs across breeds (B-DMRs), sexes (S-DMRs) and tissues (T-DMRs; see Supplementary Methods ). The high correlattion (average Pearson's r =0.994) between the number of DMRs, the number of CpGs in DMRs and the length of DMRs implied that DMR detection in regions of different length and its embeded number of CpGs was non-biased. The number of DMRs varied considerably between categories (for example, 387 muscle S-DMRs versus 218,623 muscle B-DMRs; Table 1 ). Table 1 Summary of DMRs. Full size table A macroscopical display of DMRs along chromosomes shows that DMR-rich regions also predominantly have higher CpG o/e ratios (~0.35) than the genomic average (0.21; Fig. 4a ). Over 20% of DMRs are located in subtelomeric regions, which only occupy 11.76% of the whole genome. Among the 282 pig genes that were orthologs to known human obesity-related genes [2] , [12] , [13] , [21] , 223 (~80%) were within our defined DMRs ( Fig. 4a ; Supplementary Data 1 and 2 ), which suggested that the DMRs have high association with the known obesity-related genes and these genes may have functional roles in obesity development by ways of methylation rate changes. 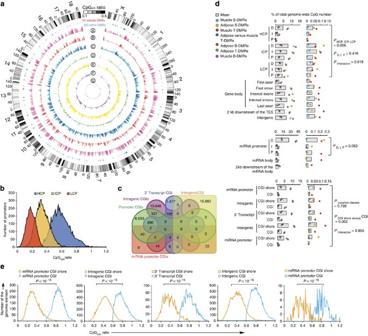Figure 4: Genome-wide distribution of differentially methylated regions. (a) Circular representation of the genome-wide distribution of DMRs. This visualisation was generated using the Circos software58. The outermost circle displays pig chromosomes with scale and the CpGo/eratio at 1 Mb bins. The second circle displays the 282 pig genes that are orthologs to the well-annotated human obesity-related genes (Supplementary Data 1), of which 223 (79%) genes overlapping the defined DMRs are in blue colour and the remaining 59 genes (21%) in red (Supplementary Data 2). The third to ninth circles represent seven categories of DMRs (A: Muscle B-DMRs, B: Adipose T-DMRs, C: Adipose B-DMRs, D: Adipose versus muscle T-DMRs, E: Muscle T-DMRs, F: Adipose S-DMRs and G: Muscle S-DMRs). The height of the histogram bins indicates number of CpGs in the DMRs. The DMR-rich (deep colour,χ2-test,P<0.001) and DMR-poor (light colour,χ2-test,P>0.001) bins are defined by comparing with genome average. TES: transcription end site. (b) All 17,930 promoters in the pig genome were classified into three types based on CpG representation. HCPs (blue,n=7,249), ICPs (yellow,n=6,629) and LCPs (red,n=4,052). (c) Venn diagram showing the distribution of all 38,778 CGIs in the pig genome among 5 CGI classes. Promoter CGIs (n=7,126), intragenic CGIs (n=13,611), 3′-transcript CGIs (n=2,305), intergenic CGIs (n=16,954) and miRNA promoter CGIs (n=169) were defined according to their genomic locations. There are overlaps between five classes of CGIs, because of the overlapping gene annotation at a specific genome coordinate. (d) Percentage of CpGs within DMRs in each of the 31 genomic elements. The statistical significance of comparison among the three miRNA promoters (D, I, P) was calculated by one-way repeated-measures ANOVA, whereas others by two-way repeated-measures ANOVA. (e) Distribution of CpGo/eratio for CGIs and their shores in five CGI classes. Wilcoxon rank-sum test was used to determine the difference of CpGo/eratio between CGIs and their shores. Figure 4: Genome-wide distribution of differentially methylated regions. ( a ) Circular representation of the genome-wide distribution of DMRs. This visualisation was generated using the Circos software [58] . The outermost circle displays pig chromosomes with scale and the CpG o/e ratio at 1 Mb bins. The second circle displays the 282 pig genes that are orthologs to the well-annotated human obesity-related genes ( Supplementary Data 1 ), of which 223 (79%) genes overlapping the defined DMRs are in blue colour and the remaining 59 genes (21%) in red ( Supplementary Data 2 ). The third to ninth circles represent seven categories of DMRs (A: Muscle B-DMRs, B: Adipose T-DMRs, C: Adipose B-DMRs, D: Adipose versus muscle T-DMRs, E: Muscle T-DMRs, F: Adipose S-DMRs and G: Muscle S-DMRs). The height of the histogram bins indicates number of CpGs in the DMRs. The DMR-rich (deep colour, χ 2 -test, P <0.001) and DMR-poor (light colour, χ 2 -test, P >0.001) bins are defined by comparing with genome average. TES: transcription end site. ( b ) All 17,930 promoters in the pig genome were classified into three types based on CpG representation. HCPs (blue, n =7,249), ICPs (yellow, n =6,629) and LCPs (red, n =4,052). ( c ) Venn diagram showing the distribution of all 38,778 CGIs in the pig genome among 5 CGI classes. Promoter CGIs ( n =7,126), intragenic CGIs ( n =13,611), 3′-transcript CGIs ( n =2,305), intergenic CGIs ( n =16,954) and miRNA promoter CGIs ( n =169) were defined according to their genomic locations. There are overlaps between five classes of CGIs, because of the overlapping gene annotation at a specific genome coordinate. ( d ) Percentage of CpGs within DMRs in each of the 31 genomic elements. The statistical significance of comparison among the three miRNA promoters (D, I, P) was calculated by one-way repeated-measures ANOVA, whereas others by two-way repeated-measures ANOVA. ( e ) Distribution of CpG o/e ratio for CGIs and their shores in five CGI classes. Wilcoxon rank-sum test was used to determine the difference of CpG o/e ratio between CGIs and their shores. Full size image We then looked at DMRs in the 31 categories of functional genomic elements. We separated promoters into three types according to the CpG representation as previously described [22] ( Fig. 4b ), and also classified CpG islands (CGIs) into five classes according to their genomic locations as previously described [23] (see Methods ; Fig. 4c ). DMRs occur more frequently in intermediate CpG promoter (ICP) than in high CpG promoter (HCP) and low CpG promoter (LCP) regions (two-way ANOVA, P =0.056; Fig. 4d ). The ICP class contains many weak CGIs [24] (<500 bp, have moderate CpG richness and/or have a GC content below 55%). This result validated previous findings that weak CGIs are more predisposed to regulation by DNA methylation and preferential targeting of weak CGIs is a general phenomenon in mammals [22] . Promoter hypermethylation has a critical role in suppressing gene expression, yet in gene bodies, it is also important in regulating alternative promoters and preventing spurious transcription initiation [23] . Interestingly, the first exon regions have the lowest DMRs within the gene body ( Fig. 4d ), which may be because of some functional motifs overlapping between the proximal region of promoters and first exons. In addition, the distal (D) regions of both mRNA and microRNA (miRNA) promoters have more DMRs than the intermediate (I) and proximal (P) regions ( Fig. 4d ), suggesting that changes in methylation at D regions of promoters may be a more prevalent mechanism for producing transcriptional variability. We found that most DMRs are located in CGI shores rather than in CGIs ( Fig. 4d ) in all five classes of genomic elements (two-way ANOVA, P =0.002), which is consistent with previous reports [25] , [26] , [27] . CpG o/e ratio of most CGI shores is around 0.35–0.36, whereas CGIs have CpG o/e ratios far greater than this cutoff (Wilcoxon rank-sum test, P <10 −16 ; Fig. 4e ), as shown by the plot of reads distribution against CpG o/e ratio in Fig. 3c . Promoter methylation and transcriptional repression We explored the correlation between methylation rate in promoters and expression level of associated mRNAs and miRNAs ( Fig. 5 ; Supplementary Fig. S4 ). It is believed that DNA methylation in promoters is only one of the several mechanisms for regulating gene expression; hence, it is logical that not all genes have correlated methylation and expression patterns. The order of correlation level in mRNA promoters, from high to low, was HCP, ICP, LCP and P, I, D ( Fig. 5 ), which validated previous report [28] . Nonetheless, as DMRs are enriched in ICPs and D regions of promoters ( Fig. 4d ), there were more mRNA-DMR pairs exhibiting correlation in ICP (8,257) than in HCP (6,217) and LCP (3,099), and more pairs in the D region (9,313) than in the I (4,923) and P (3,337) regions ( Fig. 5 ). Further, it indicated that the CpG content difference of promoters has a more profound impact on mRNA expression (two-way ANOVA, P =5.56×10 −4 ) than the distance to transcription start site (TSS) of the regions in promoters (two-way ANOVA, P =0.07). 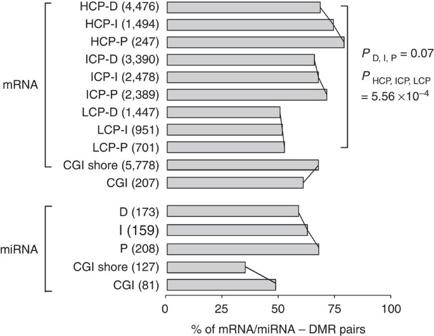Figure 5: Percentage of mRNAs and miRNAs having expression level negatively correlated with promoter methylation level. Only 3,074 probes uniquely representing 3,074 mRNA and 611 uniquely mapped miRNA genes with the high-confidence expression data from the same samples for MeDIP-seq were used (seeSupplementary Methods). The mRNA/miRNA–DMR pairs, which have downregulation together with promoter hypermethylation, or upregulation together with promoter hypomethylation, were taken as having negative correlation between expression and methylation. The total number of identified mRNA/miRNA–DMR pairs were shown in the brackets. Grey bars represent the percentage of mRNA/miRNA–DMR pairs that exhibit the inverse relationship in total mRNA/miRNA–DMR pairs. The statistical significance was calculated by two-way non-repeated-measures ANOVA. Figure 5: Percentage of mRNAs and miRNAs having expression level negatively correlated with promoter methylation level. Only 3,074 probes uniquely representing 3,074 mRNA and 611 uniquely mapped miRNA genes with the high-confidence expression data from the same samples for MeDIP-seq were used (see Supplementary Methods ). The mRNA/miRNA–DMR pairs, which have downregulation together with promoter hypermethylation, or upregulation together with promoter hypomethylation, were taken as having negative correlation between expression and methylation. The total number of identified mRNA/miRNA–DMR pairs were shown in the brackets. Grey bars represent the percentage of mRNA/miRNA–DMR pairs that exhibit the inverse relationship in total mRNA/miRNA–DMR pairs. The statistical significance was calculated by two-way non-repeated-measures ANOVA. Full size image There was correlation between miRNA expression and methylation rate in P regions of miRNA promoters (Pearson's r =−0.368, P =4.44×10 −8 ), but almost no correlation in I (Pearson's r =−0.116, P =0.146) and D (Pearson's r =0, P =0.996) regions of miRNA promoters ( Supplementary Fig. S4 ). Primary miRNA transcripts can be several thousand bases long and embeds a ~70 nucleotide long stem-loop precursor (pre-miRNA) [29] . Although little is known about the TSS of primary miRNA transcripts [30] , the results here suggested that DNA methylation in 5′ upstream of pre-miRNAs could have a role in transcriptional silencing of mature miRNA. Methylation in CGI shores had stronger (Pearson's r =−0.146, P =6.15×10 −29 ) correlation with mRNA expression than in CGIs (Pearson's r =−0.128. P =0.066; Supplementary Fig. S4 ), which is consistent with previous studies [25] , [26] , [27] . Nonetheless, miRNA expression has little or no correlation with CGI (Pearson's r =−0.133, P =0.241) and CGI shore methylation (Pearson's r =0.099, P =0.268). A recent study also showed that a common feature of DNA methylation-repressed miRNAs is the absence of CGIs in the promoter region [31] . Promoter DMRs best discriminate breeds and tissues To analyse whether DMRs exhibit any breed, sex and/or anatomic locations specific pattern, we performed unsupervised clustering for all samples using DMRs of each category of genomic elements. The adipose and muscle B-DMRs in promoters were well clustered by breed ( Fig. 6a,b ). Clustering of samples by corresponding mRNA expression is generally similar ( Supplementary Fig. S5 ), indicating consistent relationships between DNA methylation in the promoters and gene expression. The clustering by B-DMRs in CGI shores can group most samples from each breed, but not as distinctly as that by B-DMRs in promoters. This suggested that, although methylation in CGI shores is important in regulating gene expression [25] , [26] , [27] , methylation differences at promoters are better predictors of differences among the breeds. The clustering by B-DMRs of other genomic elements is even less distinct, suggesting that most methylation in these genomic elements may have weak or no direct association with functional divergence of the three breeds. 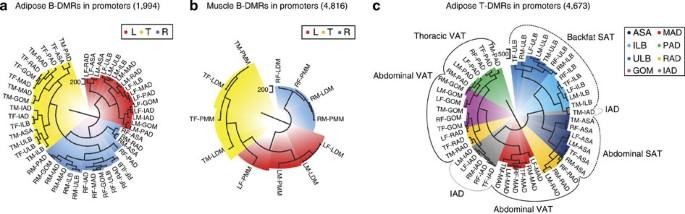Figure 6: Hierarchical clustering of samples using DMRs in promoters. (a) Clustering of adipose samples using 1,994 adipose B-DMRs in promoters. (b) Clustering of muscle samples using 4,816 muscle B-DMRs in promoters. By definition, the three pig breeds are completely segregated. The three major subgroups in the radial dendrograms correspond perfectly to pig breed, regardless of sexes and tissue types. (c) Clustering of adipose samples using 4,673 adipose T-DMRs in promoters results in most of the eight variant adipose samples are discriminated from each other. The numbers in the brackets showed the amount of DMRs used in clustering. Figure 6: Hierarchical clustering of samples using DMRs in promoters. ( a ) Clustering of adipose samples using 1,994 adipose B-DMRs in promoters. ( b ) Clustering of muscle samples using 4,816 muscle B-DMRs in promoters. By definition, the three pig breeds are completely segregated. The three major subgroups in the radial dendrograms correspond perfectly to pig breed, regardless of sexes and tissue types. ( c ) Clustering of adipose samples using 4,673 adipose T-DMRs in promoters results in most of the eight variant adipose samples are discriminated from each other. The numbers in the brackets showed the amount of DMRs used in clustering. Full size image The B-DMRs in promoters of ATs showed that the Rongchang and Tibetan breed are closer to each other than the Landrace pig ( Fig. 6a ). The same analysis in muscle tissues showed that the Landrace breed is closer to the Tibetan than the Rongchang breed ( Fig. 6b ). The same distance relationship pattern of the three breeds is reflected by the corresponding mRNA expression data clustering ( Supplementary Fig. S5 ). The different clustering patterns may be explained by the marked phenotypic changes between the feral Tibetan, the leaner Landrace and the fatty Rongchang pig breeds because of opposite breeding direction, which results in differences not only at the genetic level, but also in the epigenetic state, and potential genotype–epigenotype interactions [32] as well. In addition, the T-DMRs in promoters could largely cluster samples of the same tissue type together ( Fig. 6c ), indicating that promoter methylation also correlates with adipose distribution across the anatomic locations. It is well established that VATs have intrinsic features distinct from SATs, and are more highly correlated with the metabolic risk factors of obesity than SATs [4] , [6] , [7] , [8] . Interestingly, intermuscular adipose (IAD), which deposited between muscle bundles, was more similar to VATs in terms of methylation. This observation suggests that IAD may be a new risk factor for obesity-related diseases. Pericardial adipose (PAD) around coronary arteries is a higher correlative risk factor for cardiovascular disease than other VATs, and although thoracic PAD shares a common embryonic origin with other abdominal VATs—the splanchnic mesoderm [33] , we observed significant-site specific differences in methylation rate between them ( Fig. 6c ). Tissue types are also better discriminated by T-DMRs in promoters than in other genomic elements ( Supplementary Fig. S5 ). X chromosome methylation between male and female is expected to be significant because of the overriding effect of X chromosome inactivation in females [18] . Clustering of S-DMRs by sex was less distinct after removing DMRs on the X chromosome ( Supplementary Fig. S5 ). Genes involved in phenotypic divergence To study the association of differential methylation in promoter regions with phenotypic divergence, we first investigated the relationship between DNA methylation at promoters and the expression data of known obesity-related genes obtained through and MassArray and quantitative PCR (q-PCR). For example, FTO (fat mass- and obesity-associated gene) is a gene unequivocally associated with obesity and is ubiquitously expressed [34] , [35] . From the leaner Landrace, feral Tibetan to the fatty Rongchang breed, and across both adipose and muscle tissue types, FTO is hypermethylated in the D region of the promoter with a lower gene expression level ( Fig. 7a ). The fact that the level of methylation is highest in Landrace pig and lowest in Rongchang pig is consistent with the observation that loss of FTO expression and/or function protects against obesity and food intake [35] . ATP1B1 , which encodes the ubiquitously expressed β subunit of Na + /K + ATPase, is required for the proper cellular positioning of ATPase and its stability. Decreased ATPase activity precedes obesity and hyperinsulinaemia by influencing thermogenesis and energy balance [36] . COL8A2 , which encodes the α2 chain of type VIII collagen, is necessary for mesangial matrix expansion, as well as for hypercellularity. Lack of COL8A2 confers renoprotection in diabetic nephropathy [37] . Both ATP1B1 and COL8A2 have hypermethylation in I region of promoter and lower gene expression level that is more pronounced in the VATs and IAD than SATs ( Fig. 7b ), suggesting that hypermethylation in promoters of these two genes are potential biomarkers of high-risk visceral obesity. 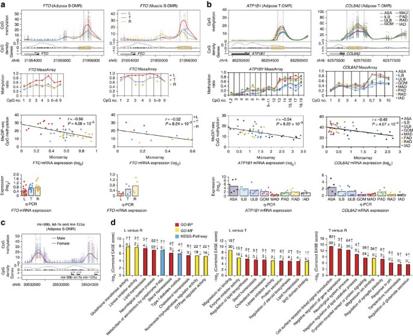Figure 7: Examples of obesity-related genes and functional gene categories showing differential DNA methylation in promoters. (a) The adipose and muscle B-DMR inFTOpromoter. Top panels, top half: CpG methylation. Each point represents methylation level (MeDIP-seq read depth) of a sample at a given CpG site. The curves showed average over the samples. The two vertical dashed lines marked the boundaries of the DMR identified. Lower half: CpG dinucleotides (black tick marks on X axis), CpG density (grey line), TSS (black arrow), exons and introns (filled black and white boxes, respectively). Plus and minus marks denote sense and antisense gene transcription. Second panels: validation of individual CpG methylation by MassArray (mapping to yellow box in upper panel). Third panels: a scatter plot and trend line (Pearson correlation) showing correlation between the log2ratios of mRNA expression from microarray and CpG methylation of the DMR from MeDIP-seq. Bottom panels: validation of mRNA expression levels by q-PCR. Bars represent the mean expression level. (b) The adipose T-DMR inATP1B1andCOL8A2promoters. (c) The adipose S-DMR in miRNAs mir-99b, let-7e and mir-125a promoters. (d) Top ten GO (Gene Ontology) and pathway categories enriched for adipose B-DMRs in promoters. The enrichment analysis was performed using the DAVID software59(seeSupplementary Methods). The EASE score, indicating significance of the comparison, was calculated using Benjamini-corrected modified Fisher's exact test. BP: biological process, MF: molecular function. Figure 7: Examples of obesity-related genes and functional gene categories showing differential DNA methylation in promoters. ( a ) The adipose and muscle B-DMR in FTO promoter. Top panels, top half: CpG methylation. Each point represents methylation level (MeDIP-seq read depth) of a sample at a given CpG site. The curves showed average over the samples. The two vertical dashed lines marked the boundaries of the DMR identified. Lower half: CpG dinucleotides (black tick marks on X axis), CpG density (grey line), TSS (black arrow), exons and introns (filled black and white boxes, respectively). Plus and minus marks denote sense and antisense gene transcription. Second panels: validation of individual CpG methylation by MassArray (mapping to yellow box in upper panel). Third panels: a scatter plot and trend line (Pearson correlation) showing correlation between the log 2 ratios of mRNA expression from microarray and CpG methylation of the DMR from MeDIP-seq. Bottom panels: validation of mRNA expression levels by q-PCR. Bars represent the mean expression level. ( b ) The adipose T-DMR in ATP1B1 and COL8A2 promoters. ( c ) The adipose S-DMR in miRNAs mir-99b, let-7e and mir-125a promoters. ( d ) Top ten GO (Gene Ontology) and pathway categories enriched for adipose B-DMRs in promoters. The enrichment analysis was performed using the DAVID software [59] (see Supplementary Methods ). The EASE score, indicating significance of the comparison, was calculated using Benjamini-corrected modified Fisher's exact test. BP: biological process, MF: molecular function. Full size image We also found correlation between methylation in promoter and gene expression, and reasonable association to breed and anatomic location divergence, for many other genes with known roles in adipose deposition and muscle growth. For example, ESD that increases expression in obesity-prone models [38] ; PPP1R3C that functions against intramyocellular lipid build-up, and reduces circulating leptin and triglycerides [39] ; GHSR that promotes growth hormone-release and increased lean, but not fat, mass in obese subjects [40] ; LIPA that inhibits intramuscular lipid stores [41] ; MC4R that inhibits food intake and prevents hyperinsulinaemia and hyperglycinaemia [42] ; and PROX1 that prevents lymphatic vascular defects that cause adult-onset obesity [43] ( Supplementary Fig. S6 ). The genes preferentially expressed in adipose (such as HEXB and HTR2A ) or muscle (such as ACE , PRKAR1A and PRKCQ ) tissues only, were validated by the methylation in the promoter and gene expression data as well ( Supplementary Fig. S6 ). The full list of candidate obesity-related genes we collected together with their DNA methylation pattern in promoters is provided in Supplementary Data 1 and 2 . In addition, out of the 2,311 genes/~282.57 Mb quantitative trait loci (QTLs) region assembled from 901 high confidence and narrowed (<2 Mb) QTLs affecting fatness and pork quality in the PigQTL database [44] ; 1,669 (72.22%) genes overlap with the defined DMRs ( Supplementary Data 3 , 4 , 5 ). This high consistency highlights the potential of identifying candidate regions or genes of quantitative traits (such as obesity) based on genome-wide DNA methylation data, such as the newly developed methylation QTL analysis [15] . Notably, out of 77 putative genes located in these QTLs region, 66 (85.71%) overlap with our defined DMRs. Methylation level of these gene's promoters strongly inversely correlated with the gene expression, suggesting that these uncharacterised protein coding genes may be involved in adipose deposition and muscle growth. Typical examples are shown in Supplementary Fig. S7 . Furthermore, numerous miRNAs having known or potential roles in obesity were also identified ( Supplementary Data 6 ). We found an S-DMR with hypermethylation in males compared with females. This S-DMR is located in the promoter region of an miRNA cluster that includes adjacent miR-99b, let-7e and miR-125a ( Fig. 7c ). Although no previous evidence exists for a direct relationship of these three miRNAs to obesity, the key functions and targets of these miRNAs are associated with the suppression of prostate cancer in male [45] and breast cancer in female [46] , and therefore, potentially contribute to sexual differences in obesity development. To identify novel genes potentially responsible for phenotypic differences, we performed enrichment analysis for genes with DMRs in promoters ( Supplementary Fig. S8 ; Supplementary Data 7 and 8 ). As expected, most enriched functional Gene Ontology categories of adipose B-DMRs in promoters were related to the pathogenesis of obesity, such as 'homeostasis of sterol, lipid, cholesterol', 'lipase inhibitor activity', 'type I diabetes mellitus' and 'dyslipidaemia' ( Fig. 7d ). Notably, the multigene family of glutathione transferase and cytochrome P450, two important groups of multifunctional detoxifying enzymes responsible for metabolising an array of xenobiotic compounds [47] , [48] , were among the enriched adipose B-DMRs in promoters ( Fig. 7d ). 'Trans-1,2-dihydrobenzene-1,2-diol dehydrogenase activity' enzymes, which also participate in metabolism of endocrinally disruptive xenobiotics [49] , were universally identified among enriched adipose T-DMRs in promoters ( Supplementary Data 8 ). Pigs as well as humans are exposed to an increasing numbers of environmental xenobiotics through ingestion of contaminated food or water, inhalation of polluted air or even dermal exposure. A link between exposure to endocrinally disruptive xenobiotics and obesity has been proposed [50] . Our finding suggests that DNA methylation rate changes of genes coding for detoxifying enzymes induced by pollutants may potentially explain the pathogenicity of obesity caused by chemical environmental endocrine disruptors. Our analyses also revealed many other functional gene categories that were potentially involved in adipose and muscle regulation ( Supplementary Data 8 ). For example, immune-related gene categories, including 'RIG-I-like receptor signalling pathway', 'interferon-α/β receptor binding', 'natural killer cell-mediated cytotoxicity' and 'antigen processing and presentation', were identified among the enriched muscle B-DMRs in promoters, which is consistent with previous finding of obesity-induced immune dysfunction [51] . Intriguingly, given that AT derives from mesoderm, the identification of 'mesoderm development' gene category among enriched adipose S-DMRs in promoters indicated that sex-specific obesity is potentially related to the establishment of differential methylation during embryonic development. In addition, the enriched gene categories of muscle T-DMRs, and adipose versus muscle T-DMRs, in promoters reflected the well-characterised tissue-specific functions. Methylation differences in genes coding for proteins involved in GTP-related energy metabolism may be responsible for the differences in percentage of mitochondria between the two phenotypically distinct SMTs [17] . Differential methylation of genes involved in 'cytoskeletal protein binding', 'regulation of cellular protein metabolic process' and 'enzyme activator activity' may explain the developmental differences between adipose and muscle tissues [52] . This study reports the comprehensive genome-wide epigenetic survey of various adipose and SMTs, based on directly sequenced animal DNA methylomes. Through identification of DMRs among breeds, sexes and anatomic locations, and classification of the DMRs according to their locations in various genomic elements, we found that DMRs in promoters can repress gene expression and are highly associated with phenotypic variation. Identified DMRs were preferentially situated in ICP and in CGI shores. This validated the hypothesis that weak CGIs are more prone to regulation by DNA methylation, as the higher feasibility for weak CGIs to become de novo methylated regions, and preferentially associated with the general phenomenon and non-malignant, common complex diseases (such as obesity) instead of the highly heterogeneous lesions (such as cancer) [22] . We also found that the intermuscular IAD was more similar to the VATs in methylation pattern, which provided the first epigenomic evidence for IAD as a candidate risk factor for obesity. The data set and research here shed new light on the epigenomic regulation of adipose deposition and muscle growth. It is considered that pigs can serve as a good biomedical model for human obesity studies because they share the same general physiology with human. Indeed, we found that about 80% of the known or candidate human obesity-related genes and 72% of genes in the QTL regions that affect fatness and pork quality were within our defined DMRs. Detailed analysis indicated that the methylation regulation patterns of these genes are consistent with their known biological functions. We also predicted many novel candidate genes that were associated with variation in obesity-related phenotypes and that require further experimental validation. Domesticated breeds also provide additional advantage of highly homogeneous genetic backgrounds, large litter size (10~12 piglets per litter; 24~36 piglets per year), short generation interval (12 months) and a homogeneous feeding regime, which are particularly suitable for survey of transgenerational epigenetic inheritance [53] . In addition to providing new information for biomedical research, genomic/epigenomic studies of pigs may also help uncover the molecular basis that underlies economic traits in pig, which can be used to improve the efficiency of artificial selection, hence the production of healthier pork. Animals Nine females and nine males at 210-day-old for each of the Landrace (a leaner, Western breed), the Tibetan (a feral, indigenous Chinese pig that has not undergone artificial selection) and the Rongchang (a fatty, Chinese breed) pig breeds were used in this study. There is no direct and collateral blood relationship within the last 3 generations among the 18 pigs from each of the breeds. The piglets were weaned simultaneously at 28±1 day of age. A starter diet provided 3.40 Mcal kg −1 metabolisable energy (ME), 20.00% crude protein and 1.15% lysine from the thirtieth to sixtieth day after weaning. From the sixty-first to one hundred and twentieth day, the diet contained 3.40 Mcal kg −1 ME, 17.90% crude protein and 0.83% lysine. From the one hundred and twenty-first to two hundred and tenth day, the diet contained 3.40 Mcal kg −1 ME, 15.00% crude protein and 1.15% lysine. The animals were allowed access to feed and water ad libitum and lived under the same normal conditions. Tissue collection Animals were humanely killed as necessary to ameliorate suffering and not fed the night before they were slaughtered. All the animals and samples used in this study were collected according to the guidelines for the care and use of experimental animals established by the Ministry of Agriculture of China. Eight ATs from different body sites and two phenotypically distinct SMTs were rapidly separated from each carcass, immediately frozen in liquid nitrogen and stored at −80 °C until RNA and DNA extraction. The eight ATs are divided into four groups: (1) three types of SATs (that is, abdominal subcutaneous adipose, upper layer of backfat and inner layer of backfat near the last third or fourth rib); (2) three types of VATs in the abdominal cavity (i.e., greater omentum, mesenteric adipose and retroperitoneal adipose); (3) one type of VAT in the thoracic cavity (i.e., PAD, which is located between visceral and parietal pericardium); and (4) IAD, the adipose visible between muscle groups and beneath the muscle fascia in the hips. Two phenotypically distinct SMTs are LDM (typical white SMT) near the last third or fourth rib and the intermediate section of PMM (typical red SMT). Measurements of obesity-related phenotype Measurements of pig body density, concentrations of 24 serum-circulating indicators of metabolism, adipocyte volume, myofibre cross-sectional area, myofibre type rate (fast/slow) and fatty acid composition are described in detail in Supplementary Methods . Methylated DNA immunoprecipitation sequencing We randomly selected three pigs with a specific sex from each breed as biological replicates. And we have ten tissues for each individual; so in total, 180 samples were sequenced separately. MeDIP DNA libraries were prepared following the protocol as our previous description [54] . Each MeDIP library was subjected to paired-end sequencing using Illumina HiSeq 2000 and a 50 bp read length. Details are listed in Supplementary Methods . Identification of DMRs After filtering the low-quality reads, the MeDIP-seq data were aligned to the UCSC pig reference genome (Sscrofa9.2) using SOAP2 (Version 2.21) [55] . The genomic regions enriched in methylated CpGs B-DMRs, S-DMRs and T-DMRs were identified using our newly developed method by calculating variation of single CpG. Additional details for the process are listed in Supplementary Methods . Definition of genomic elements We referred to the UCSC pig reference genome (Sscrofa9.2) annotation data for the identification of genomic elements. All 17,930 promoters (−2,200 to +500 bp) were classified into three types according to CpG representation as previously described [22] . There were 7,249 HCPs, 6,629 ICPs and 4,052 LCPs ( Fig. 4b ). Each promoter of 2,700 bp length was divided into three regions as previously described [28] : P (−200 to +500 bp), I (−200 to −1,000 bp) and D (−1,000 to −2,200 bp). We obtained genomic locations of 38,778 CGIs and definitions of 21,533 Ensembl genes from the UCSC pig reference genome (Sscrofa9.2), as well as genomic locations of 803 pre-miRNAs based on our small RNA-seq results. We grouped CGIs into five classes on the basis of their distance to Ensembl genes or pre-miRNAs as previously described [23] with some modifications ( Fig. 4c ). There are (1) 7,126 promoter CGIs (if a CGI ends after 1,000 bp upstream of a gene's TSS, and starts before 300 bp downstream of a gene's TSS); (2) 13,611 intragenic CGIs (if a CGI starts after 300 bp downstream of a gene's TSS and ends before 300 bp upstream of a gene's transcription end site (TES)); (3) 2,305 3′-transcript CGIs (if a CGI ends after 300 bp upstream of a gene's TES and starts before 300 bp downstream of a gene's TES); (4) 16,954 intergenic CGIs (if a CGI starts after 300 bp downstream of a gene's TES and ends before 1,000 bp upstream of a gene's TSS); (5) 169 miRNA promoter CGIs (if there was a >60% overlap of a CGI with 2 kb upstream of the pre-miRNA). There are overlaps between five classes of CGIs, because of the overlapping gene annotation at a specific genome coordinate. CGI shores were defined as extending up to 2 kb from CGIs. We also identified the genomic locations of the 17,932 first exons, 14,760 first introns, 117,200 internal exons, 116,186 internal introns and 15,259 last exons of the 21,533 Ensembl genes, together with the 13,626 intergenic regions, 4,309,043 repeats and 59,385 SNPs by referring to the UCSC Genome Browser for pig. MassArray The DNA isolated from three biological replicates for each breed/sex/tissue type combination were pooled in equal quantities and treated with bisulphite using an EZ DNA methylation-Gold Kit (ZYMO Research) according to the manufacturer's specifications. Quantitative methylation analysis of the DMRs was performed using the Sequenom MassARRAY platform (CapitalBio, Beijing, China) as described previously [56] . PCR primers were designed using the EpiDesigner software (Sequenom). The oligo sequences and the genomic coordinates of the amplicons across which DNA methylation was assessed in this study are given in Supplementary Table S2 . The resultant methylation calls were analysed with EpiTyper software v1.0 (Sequenom) to generate quantitative results for each CpG or an aggregate of multiple CpGs. Gene expression microarray Genome-wide gene expression analysis of 180 samples that corresponded to the samples used for MeDIP-seq was performed using the Agilent Pig Gene Expression Oligo Microarray (Version 2). Data analysis was performed with MultiExperiment Viewer. Details are listed in Supplementary Methods . Quantitative PCR RNase-free DNase I (TaKaRa) was used for removal of genomic DNA from RNA samples used for microarray analysis. cDNA was synthesised using the oligo (dT) and random 6-mer primers provided in the PrimeScript RT Master Mix kit (TaKaRa). q-PCR was performed using the SYBR Premix Ex Taq kit (TaKaRa) on a CFX96 Real-Time PCR detection system (Bio-Rad). Primer sequences used for the q-PCR are shown in Supplementary Table S3 . All measurements contained a negative control (no cDNA template), and each RNA sample was analysed in triplicate. Porcine ACTB , TBP and TOP2B were simultaneously used as endogenous control genes. Relative expression levels of objective mRNAs were calculated using the ΔΔCt method. miRNA discovery and profiling Eight ATs and two SMTs of the three female Landrace pigs were used for small RNA-seq. The construction of small RNA libraries and single-end sequencing in 36 bp reads using Illumina Genome Analyzer II, generated a total of 7.12 Gb reads for the ten libraries. The bioinformatics pipeline for miRNA discovery was carried out as our previous description [57] , with some improvements. Details are listed in Supplementary Methods . Our results extend the repertoire of pig miRNAome to 803 pre-miRNAs (174 known, 210 novel and 419 candidate), encoding for 1,014 mature miRNAs, of which 952 are unique ( Supplementary Data 9 ). Acccession codes: The high-throughput sequencing data and microarray data have been deposited in NCBI's Gene Expression Omnibus under GEO Series accession numbers GSE30344 (MeDIP-seq data), GSE30343 (gene expression microarray data) and GSE30334 (small RNA-seq data). How to cite this article: Li, M. et al . An atlas of DNA methylomes in porcine adipose and muscle tissues. Nat. Commun. 3:850 doi: 10.1038/ncomms1854 (2012).